A system for the continuous directed evolution of proteases rapidly reveals drug-resistance mutations The laboratory evolution of protease enzymes has the potential to generate proteases with therapeutically relevant specificities and to assess the vulnerability of protease inhibitor drug candidates to the evolution of drug resistance. Here we describe a system for the continuous directed evolution of proteases using phage-assisted continuous evolution (PACE) that links the proteolysis of a target peptide to phage propagation through a protease-activated RNA polymerase (PA-RNAP). We use protease PACE in the presence of danoprevir or asunaprevir, two hepatitis C virus (HCV) protease inhibitor drug candidates in clinical trials, to continuously evolve HCV protease variants that exhibit up to 30-fold drug resistance in only 1 to 3 days of PACE. The predominant mutations evolved during PACE are mutations observed to arise in human patients treated with danoprevir or asunaprevir, demonstrating that protease PACE can rapidly identify the vulnerabilities of drug candidates to the evolution of clinically relevant drug resistance. Among the more than 600 naturally occurring proteases that have been described [1] are enzymes that have proven to be important catalysts of industrial processes, essential tools for proteome analysis and life-saving pharmaceuticals [2] , [3] , [4] , [5] . Recombinant human proteases including thrombin, factor VIIa, and tissue plasminogen activator are widely used drugs for the treatment of blood clotting diseases [4] . In addition, the potential of protease-based therapeutics to address disease in a manner analogous to that of antibody drugs [6] , [7] , but with catalytic turnover, has been recognized for several decades [4] , [8] . Natural proteases, however, typically target only a narrowly defined set of substrates, limiting their therapeutic potential. The directed evolution of proteases in principle could generate enzymes with tailor-made specificities, but laboratory-evolved proteases are frequently non-specific, weakly active or only modestly altered in their substrate specificity, limiting their utility [9] , [10] , [11] , [12] , [13] , [14] . In addition to their importance as current and future therapeutic agents, proteases have also proven to be major drug targets for diseases including cardiovascular illness, infectious disease and cancer [15] , [16] . While drug specificity and potency are characterized and optimized during pre-clinical studies, the evolution of drug resistance is often not well understood until it arises in patients, despite the strong relationship between drug resistance vulnerability and a lack of therapeutic efficacy. For example, resistance to HIV and HCV protease inhibitors can arise in as few as 2 days of clinical use [17] and frequently leads to viral rebound and poor treatment outcomes [18] , [19] , [20] , [21] . The speed with which drug resistance can arise in the clinic endangers patients and puts years of drug development efforts before such a determination at risk. Unfortunately, characterizing the potential of protease inhibitors to be overcome by the evolution of drug resistance using methods such as mammalian cell culture, animal models or yeast display-based laboratory evolution is time- and labor-intensive [22] , [23] . As a result, identifying drug resistance vulnerabilities of early-stage preclinical candidates is not a common practice. Phage-assisted continuous evolution (PACE) in principle could serve as a rapid, high-throughput method to evolve protease enzymes and to reveal resistance to protease inhibitor drug candidates, analogous to previous uses of stepwise protein evolution to study antibiotic resistance [24] . During PACE, continuously replicating M13 bacteriophage in a fixed-volume vessel (a ‘lagoon’) carries an evolving gene of interest. Phage with genes encoding proteins with the desired target activity preferentially replicate because target activity triggers the production of pIII, an essential component in the bacteriophage life cycle [25] . Because the lagoon is continuously diluted by a constant influx of host E. coli cells, phage encoding inactive variants produce non-infectious progeny that are rapidly diluted out of the lagoon. Dilution occurs faster than cell division but slower than phage replication, ensuring that mutations only accumulate in the phage genome. Because evolution during PACE takes place continuously without researcher intervention, hundreds of theoretical rounds of evolution can be performed per week. We speculated that PACE could be well suited to the directed evolution of proteases, which may require many successive mutations to remodel complex networks of contacts with polypeptide substrates [26] , [27] . Moreover, the speed of PACE may enable the rapid identification of mutations that confer resistance to protease inhibitors. To date, however, PACE has only been reported to evolve RNA polymerase enzymes [25] , [28] , [29] , [30] . Here we describe the development and application of a system for the continuous directed evolution of proteases. This system uses an engineered protease-activated RNA polymerase (PA-RNAP) to transduce polypeptide cleavage events into changes in gene expression that support phage propagation during PACE. We validate that this system successfully links the phage life cycle to protease activity for three distinct proteases. When performed in the presence of danoprevir or asunaprevir, two hepatitis C virus (HCV) protease inhibitor drug candidates currently in clinical trials, protease PACE rapidly evolved HCV protease variants that are resistant to each drug candidate. The PACE-evolved HCV protease variants are dominated by mutations previously observed in patients treated with these drug candidates. Together, these findings establish a new platform to rapidly generate proteases with novel properties through continuous evolution and to reveal the vulnerability of protease inhibitors to the evolution of drug resistance. Transducing protease activity into gene expression PACE requires that a target activity be linked to changes in the expression of an essential phage gene such as gene III (gIII). To couple the cleavage of a polypeptide substrate to increases in gene expression, we engineered a PA-RNAP that transduces proteolytic activity into changes in gene expression that are sufficiently strong and rapid to support PACE. T7 RNA polymerase (T7 RNAP) is naturally inhibited when bound to T7 lysozyme [31] . We envisioned that T7 lysozyme could be tethered to T7 RNAP through a flexible linker containing a target protease cleavage site. Ideally, the effective concentration of the tethered T7 lysozyme with respect to T7 RNAP would be sufficiently high that the T7 RNAP subunit would exist predominantly in the T7 lysozyme-bound, RNAP-inactive state. Proteolysis of the target sequence would disfavour the bound T7 RNAP:T7 lysozyme complex, resulting in the liberation of an active T7 RNAP and expression of gIII placed downstream of a T7 promoter ( Fig. 1a ). 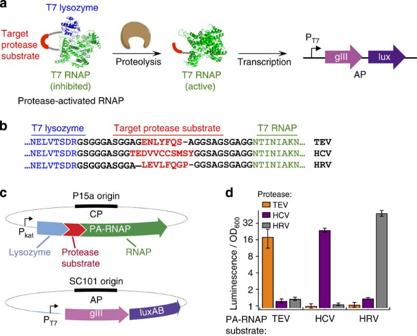Figure 1: Development of a system to link protease activity to gene expression. (a) Protease-activated RNA polymerase (PA-RNAP). T7 RNAP is fused to the natural inhibitor T7 lysozyme through a linker containing a protease target substrate sequence. While the linker is intact, the complex preferentially adopts the lysozyme-bound, RNAP-inactive state. Proteolysis of the target sequence favours dissociation of the complex, freeing active T7 RNAP to transcribe genes downstream of the T7 promoter. This study used an accessory plasmid (AP) in which the T7 promoter drives a tandem gIII-luciferase (lux) cassette. (b) Sequences of the protein linkers containing a target protease substrate used for each PA-RNAP, with T7 lysozyme residues in blue, protease substrates in red, T7 RNAP residues in green and linker regions in black. (c) Plasmids used for protease PACE. An AP that has gIII and luciferase (lux) under the control of the T7 promoter serves as the source of gIII in the cells. A complementary plasmid (CP) constitutively expresses a PA-RNAP variant with a protease target substrate sequence embedded in the linker. (d) PA-RNAP gene expression response inE. colicells. Host cells were transformed with (i) an AP containing the T7 promoter driving gIII-lux; (ii) a CP that constitutively expresses a PA-RNAP including the TEV protease substrate, the HCV protease substrate, or the HRV protease substrate; and (iii) a plasmid that expresses TEV protease (orange bars), HCV protease (purple bars), or HRV protease (grey bars). Gene expression is activated only when the expressed protease cleaves the amino-acid sequence on the PA-RNAP sensor. The luminescence experiment was performed in triplicate with error bars indicating the s.d. Figure 1: Development of a system to link protease activity to gene expression. ( a ) Protease-activated RNA polymerase (PA-RNAP). T7 RNAP is fused to the natural inhibitor T7 lysozyme through a linker containing a protease target substrate sequence. While the linker is intact, the complex preferentially adopts the lysozyme-bound, RNAP-inactive state. Proteolysis of the target sequence favours dissociation of the complex, freeing active T7 RNAP to transcribe genes downstream of the T7 promoter. This study used an accessory plasmid (AP) in which the T7 promoter drives a tandem gIII-luciferase (lux) cassette. ( b ) Sequences of the protein linkers containing a target protease substrate used for each PA-RNAP, with T7 lysozyme residues in blue, protease substrates in red, T7 RNAP residues in green and linker regions in black. ( c ) Plasmids used for protease PACE. An AP that has gIII and luciferase (lux) under the control of the T7 promoter serves as the source of gIII in the cells. A complementary plasmid (CP) constitutively expresses a PA-RNAP variant with a protease target substrate sequence embedded in the linker. ( d ) PA-RNAP gene expression response in E. coli cells. Host cells were transformed with (i) an AP containing the T7 promoter driving gIII-lux; (ii) a CP that constitutively expresses a PA-RNAP including the TEV protease substrate, the HCV protease substrate, or the HRV protease substrate; and (iii) a plasmid that expresses TEV protease (orange bars), HCV protease (purple bars), or HRV protease (grey bars). Gene expression is activated only when the expressed protease cleaves the amino-acid sequence on the PA-RNAP sensor. The luminescence experiment was performed in triplicate with error bars indicating the s.d. Full size image N-terminal fusions to T7 RNAP are known to be well tolerated, and, in the crystal structure of T7 RNAP bound to T7 lysozyme, the C terminus of T7 lysozyme is only 32 Å from the N terminus of T7 RNAP, separated by a solvent-exposed channel [32] ( Supplementary Fig. 1 ). In light of this structural information, we linked the two proteins through these proximal termini. As T7 lysozyme activity is toxic to host E. coli cells, we characterized catalytically inactive lysozyme variants and found that the inactive C131S lysozyme mutant retained its ability to inhibit T7 RNAP without impairing host cell viability. To identify T7 RNAP–T7 lysozyme linkers that promote complex formation and result in an inactive polymerase subunit yet permit efficient proteolysis, we screened a small set of linkers consisting of Gly, Ser and Ala ranging in length from 3 to 10 residues flanking each side of a target protease substrate. We designed PA-RNAP constructs containing linker peptide sequences known to be cleaved by tobacco etch virus (TEV) protease, HCV protease or human rhinovirus -14 3C (HRV) protease. We assayed T7 RNAP activity using a luciferase reporter and observed that T7 lysozyme linked to T7 RNAP through at least 28 residues including the target protease substrate resulted in significant inhibition of RNAP activity ( Fig. 1b ). To assay RNAP activation, we coexpressed each PA-RNAP variant from a plasmid (the complementary plasmid or CP, Fig. 1c and Supplementary Fig. 2 ) together with each of the three proteases (expressed from the expression plasmid or EP, Supplementary Fig. 3 ) in E. coli cells that also harboured a plasmid encoding gIII and luciferase under control of the T7 promoter (the accessory plasmid or AP, Fig. 1c and Supplementary Fig. 4 ). Expression of a protease that is not known to cleave the target amino-acid sequence in a coexpressed PA-RNAP did not result in enhanced gene expression as measured by luciferase activity ( Fig. 1d ). In contrast, expression of a protease that is known to cleave the target sequence within the PA-RNAP resulted in 18- to 49-fold increase in gene expression for all three cognate combinations of protease and substrate. These data indicate that PA-RNAPs are capable of transducing specific proteolytic cleavage activities into large changes in target gene expression. Linking protease activity to phage propagation Next we sought to use PA-RNAPs to link the life cycle of M13 bacteriophage to protease activity. We generated selection phage (SP) in which gIII was replaced by a gene encoding TEV protease, HCV protease or HRV protease ( Supplementary Fig. 5 ). Without pIII, these phage are unable to propagate on wild-type E. coli cells. We engineered host E. coli cells containing two plasmids: ( i ) an AP that contains gIII and luciferase under the control of the T7 promoter and ( ii ) a CP that constitutively expresses a PA-RNAP ( Fig. 1c ). To be sure that the PA-RNAP selection scheme work as intended we analysed the cleavage of the sensor by western blot. We observed the loss of the lysozyme-RNAP fusion and the formation of a new protein that corresponds to the size of T7 RNAP exclusively in the presence of protease phage that recognizes the host encoded PA-RNAP ( Supplementary Fig. 6 ). To assay whether the host cells could support phage propagation in a protease-dependent manner, we performed activity-dependent plaque assays. We observed that plaque formation, a consequence of phage replication in solid media, only occurred with phage encoding a protease that can cleave the PA-RNAP within the host cells. Phage with mismatched protease/PA-RNAP combinations did not form plaques, indicating that phage encoding non-cognate proteases do not replicate, or replicate at a significantly reduced rate. These observations together establish that the PA-RNAP system is capable of transducing protease activity of a phage-encoded protease into phage production. We next tested whether the PA-RNAP-based selection supports the continuous propagation of phage encoding active proteases in the continuous liquid culture format required for PACE ( Fig. 2a ). We maintained three host cell cultures, each harbouring a CP expressing a PA-RNAP containing one of the three protease cleavage sites (TEV, HCV or HRV protease substrates), using chemostats diluted with fresh growth media at a fixed rate [30] . Each of these host cell cultures continuously diluted lagoons seeded with various combinations of phage containing TEV, HCV or HRV protease. Lagoons seeded with phage encoding cognate proteases that can cleave the PA-RNAP within the host cells robustly propagated (10 8 –10 10 p.f.u. ml −1 after 72 h of continuous dilution at 1.0 lagoon volume per hour), while lagoons seeded with phage encoding proteases that do not match the PA-RNAP of incoming host cells washed out (<10 4 p.f.u. ml −1 ), demonstrating protease activity-dependent propagation in continuous liquid culture. 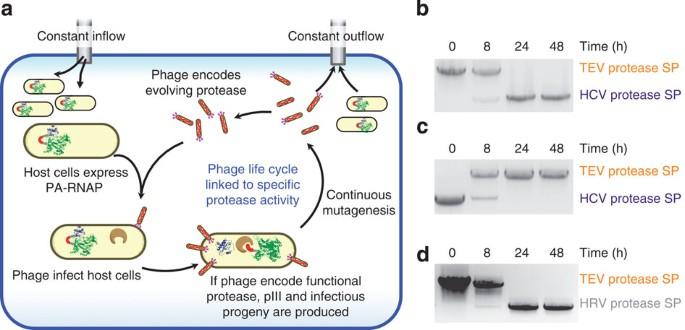Figure 2: PA-RNAPs link protease activity to phage propagation. (a) The protease PACE system. Fixed volume vessels (lagoons) contain phage in which gIII is replaced with a gene encoding an evolving protease. The lagoon is fed with host cells that contain an AP with the T7 promoter driving gIII and a CP that expresses a PA-RNAP. Phages infect incoming cells and inject their genome containing a protease variant. Only if the protease variant can activate the PA-RNAP by cleaving the linker encoding the target protease substrate, gIII is expressed and that SP can propagate. (b–d) Enrichment of active proteases from mixed populations using PACE. At time 0, a lagoon was seeded with a 1,000-fold excess of non-cognate protease-encoding phage over cognate protease-encoding phage. The lagoon was continuously diluted with host cells containing a PA-RNAP with either the HCV (b), TEV (c) or HRV (d) protease substrates. Lagoon samples were periodically analysed by PCR. In all three cases, phage encoding the cognate protease were rapidly enriched in the lagoon while phage encoding the non-cognate protease were depleted. Full gels are shown inSupplementary Fig. 8. Figure 2: PA-RNAPs link protease activity to phage propagation. ( a ) The protease PACE system. Fixed volume vessels (lagoons) contain phage in which gIII is replaced with a gene encoding an evolving protease. The lagoon is fed with host cells that contain an AP with the T7 promoter driving gIII and a CP that expresses a PA-RNAP. Phages infect incoming cells and inject their genome containing a protease variant. Only if the protease variant can activate the PA-RNAP by cleaving the linker encoding the target protease substrate, gIII is expressed and that SP can propagate. ( b – d ) Enrichment of active proteases from mixed populations using PACE. At time 0, a lagoon was seeded with a 1,000-fold excess of non-cognate protease-encoding phage over cognate protease-encoding phage. The lagoon was continuously diluted with host cells containing a PA-RNAP with either the HCV ( b ), TEV ( c ) or HRV ( d ) protease substrates. Lagoon samples were periodically analysed by PCR. In all three cases, phage encoding the cognate protease were rapidly enriched in the lagoon while phage encoding the non-cognate protease were depleted. Full gels are shown in Supplementary Fig. 8 . Full size image To determine whether this system can selectively replicate phage carrying protease genes with a desired activity at the expense of phage encoding proteases that are unable to cleave the host-cell PA-RNAP, we performed protease phage enrichment experiments in a PACE format. We seeded a lagoon with a 1,000:1 ratio of TEV SP:HCV SP, then allowed the phage to propagate in the lagoon while being continuously diluted with host cells containing a PA-RNAP with the HCV protease recognition site. We periodically sampled the waste line of the lagoon and amplified by PCR the region of the phage containing the protease genes. The TEV protease and HCV protease genes are readily distinguishable as PCR amplicons of distinct lengths. At the start of the experiment, the HCV protease phage were virtually undetectable by PCR amplification of the starting population and gel electrophoresis, while TEV protease dominated the lagoon ( Fig. 2b ). After just 24 h of continuous propagation on host cells containing the HCV PA-RNAP, the TEV protease SPs were undetectable, while the HCV protease SPs were strongly enriched (≥100,000-fold enrichment over 24 h). We repeated this experiment with a 1,000-fold excess of HCV protease phage over TEV protease phage using host cells containing the TEV protease PA-RNAP ( Fig. 2c ), and a third time using a 1,000-fold excess of TEV protease phage over HRV phage and host cells containing the HRV protease PA-RNAP ( Fig. 2d ). In all three of the enrichment experiments, continuous propagation rapidly and markedly enriched phage encoding each cognate protease from a minute fraction of the starting phage mixture, while non-cognate proteases washed out of the lagoon ( Fig. 2 ). Collectively, these results indicate that this protease PACE system successfully links specific protease activity to the phage life cycle in a continuous flow format and can strongly and rapidly enrich phage that encodes proteases with the ability to cleave a target polypeptide substrate. Continuous evolution of resistance to HCV protease inhibitors As an initial application of protease PACE, we continuously evolved protease enzymes to rapidly assess the drug resistance susceptibility of small-molecule protease inhibitors. Several HCV protease inhibitors are in late-stage clinical trials or are awaiting FDA approval [33] , [34] . For some HCV protease inhibitor drug candidates, clinically isolated drug-resistant mutations are known [20] . First we tested whether small-molecule HCV protease inhibitors can modulate protease activity in the protease PACE system. We observed that the incubation of host cells with either danoprevir (IC 50 =~0.3 nM) [35] or asunaprevir (IC 50 =~1.0 nM) [36] , two second-generation HCV protease inhibitors, inhibited the cellular gene expression arising from the activity of HCV protease on the HCV PA-RNAP in a dose-dependent manner ( Fig. 3 ). These observations suggest that protease inhibitors can create selection pressure during PACE favouring the evolution of protease mutants that retain their ability to cleave a cognate substrate despite the presence of the drug candidates. 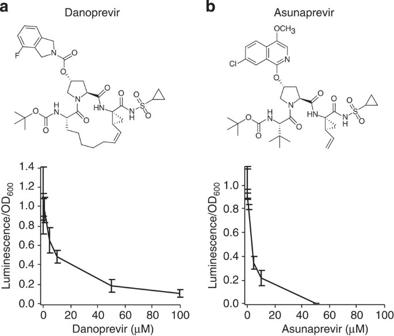Figure 3: HCV PA-RNAP response to protease inhibitors inE. colicells. Host cells expressing the HCV PA-RNAP were incubated with HCV protease inhibitors danoprevir (a) or asunaprevir (b) for 90 min, followed by inoculation with HCV protease encoding phage. After 3 h, luminescence assays were used to quantify relative gene activation resulting from the PA-RNAP. Luminescence experiments were performed in triplicate with error bars depicting the s.d. Figure 3: HCV PA-RNAP response to protease inhibitors in E. coli cells. Host cells expressing the HCV PA-RNAP were incubated with HCV protease inhibitors danoprevir ( a ) or asunaprevir ( b ) for 90 min, followed by inoculation with HCV protease encoding phage. After 3 h, luminescence assays were used to quantify relative gene activation resulting from the PA-RNAP. Luminescence experiments were performed in triplicate with error bars depicting the s.d. Full size image On the basis of the relationship between protease inhibitor concentration and gene expression in our system ( Fig. 3 ) and initial trial PACE experiments, we selected 20 μM danoprevir as the final concentration to use in the culture media during attempts to continuously evolve drug-resistant HCV proteases. We inoculated two separate lagoons with HCV protease SP and propagated the phage on host cells containing the HCV protease PA-RNAP in the absence of any inhibitor for 6 h to allow the accumulation of mutations in HCV protease genes. Next, we added 20 μM danoprevir to the media that feeds into the host cell culture, and eventually into each of the two replicate lagoons. As a control, we propagated two replicate lagoons of HCV protease phage on HCV protease PA-RNAP host cells with no added protease inhibitor for the same time period. Throughout all of these experiments, we induced enhanced mutagenesis of the phage genome by activating an improved mutagenesis plasmid (MP) in the host cells with 0.5% arabinose ( Supplementary Table 1 ). Phage populations at 6 and 28 h from replicate lagoons were analysed by high-throughput DNA sequencing. No mutations were substantially enriched in the control lagoons propagated in the absence of any drug candidate ( Fig. 4c ). In contrast, several mutations rapidly evolved in both replicate lagoons in the presence of danoprevir. Mutations at position D168 were predominant among these mutations. By 28 h, lagoon 1 with danoprevir contained 38.8% D168E, 8.3% D168Y, 2.1% D168A and 1.1% D168V, while lagoon 2 with danoprevir contained 40.3% D168E and 10.7% D168Y ( Fig. 4c ). Other genetic differences between the SPs of these two replicate populations, such as R130C (5.1% in lagoon 1, undetectable in lagoon 2) and T72I (10.8% in lagoon 2, undetectable in lagoon 1), suggest that cross-contamination did not lead to the observed protease variants in these experiments. These findings reveal that the presence of danoprevir caused the population of continuously evolving proteases to rapidly acquire mutations at D168. 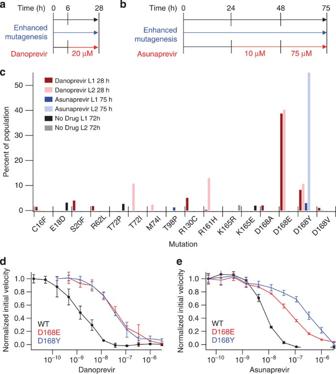Figure 4: Continuous evolution of drug resistance in HCV protease. (a,b) PACE condition timeline for evolution in the presence of danoprevir (a) or asunaprevir (b). The blue arrows indicate arabinose-induced enhanced mutagenesis, and the red arrow shows the timing and dosing of HCV protease inhibitors. (c) High-throughput sequencing data from phage populations in replicate lagoons (L1 and L2) subjected to danoprevir treatment at 28 h, asunaprevir treatment at 75 h, and no drug at 72 h. All mutations with frequencies >1% above the allele-specific error rate are shown. (d)In vitroanalysis of danoprevir inhibition of mutant HCV proteases that evolved during PACE. (e)In vitroanalysis of asunaprevir inhibition of mutant HCV proteases that evolved during PACE. For (d,e), evolved HCV protease variants were expressed and purified, then assayed using an internally quenched fluorescent-substrate (Anaspec).In vitroanalyses were performed in triplicate with error bars calculated as the s.d. Figure 4: Continuous evolution of drug resistance in HCV protease. ( a , b ) PACE condition timeline for evolution in the presence of danoprevir ( a ) or asunaprevir ( b ). The blue arrows indicate arabinose-induced enhanced mutagenesis, and the red arrow shows the timing and dosing of HCV protease inhibitors. ( c ) High-throughput sequencing data from phage populations in replicate lagoons (L1 and L2) subjected to danoprevir treatment at 28 h, asunaprevir treatment at 75 h, and no drug at 72 h. All mutations with frequencies >1% above the allele-specific error rate are shown. ( d ) In vitro analysis of danoprevir inhibition of mutant HCV proteases that evolved during PACE. ( e ) In vitro analysis of asunaprevir inhibition of mutant HCV proteases that evolved during PACE. For ( d , e ), evolved HCV protease variants were expressed and purified, then assayed using an internally quenched fluorescent-substrate (Anaspec). In vitro analyses were performed in triplicate with error bars calculated as the s.d. Full size image To assay whether the PACE-evolved mutations confer danoprevir drug resistance in HCV protease, we purified recombinant HCV protease variants containing either of the two most highly enriched mutations, D168E and D168Y. Each of these two mutations increase the IC 50 of danoprevir by ~30-fold (wild-type HCV protease IC 50 =1.3±0.1 nM; HCV protease D168E IC 50 =38.9±2.4 nM; HCV protease D168Y IC 50 =34.4±2.8 nM; IC 50 ±s.d.) ( Fig. 4d ). Importantly, the D168E, D168A and D168V mutations emerging from protease PACE have been previously identified as common drug-resistant mutations in HCV isolated from patients treated with danoprevir [20] , [37] . To validate that protease PACE in the presence of a different HCV protease inhibitor can also result in the rapid evolution of drug-resistant mutations, we repeated PACE of HCV protease in the presence of asunaprevir, an HCV protease inhibitor in phase III clinical trials, instead of danoprevir. We selected 75 μM asunaprevir as the final target concentration to use in the culture media based on dose-dependent gene expression assays ( Fig. 3 ). To allow diversity to emerge in the protease population, we first propagated HCV protease phage for 24 h without any inhibitor. Next, to ensure that the populations had sufficient time to evolve mutations that confer drug resistance, we propagated the populations for 24 h with 10 μM asunaprevir, Finally, we ramped up the asunaprevir concentration to 75 μM for 27 h to enrich those mutations that conferred robust drug resistance. HCV protease phage were also propagated for an identical amount of time without any added drug candidate for comparison. High-throughput DNA sequencing of phage populations at the end of the experiment revealed that mutations evolved at substantial levels in the asunaprevir-treated lagoons but not in the control samples ( Fig. 4c ). In this experimental condition as well, mutations at position D168 were highly enriched. In the case of asunaprevir, however, the only substitution at this position to emerge at substantial levels from protease PACE was D168Y, in contrast with the evolution of both D168E and D168Y during protease PACE with danoprevir. In vitro assays of HCV proteases containing either mutation provides an explanation underlying the strong apparent preference of D168Y over D168E within asunaprevir-treated lagoons. D168Y increases the IC 50 of asunaprevir by 30-fold, while D168E only increases the IC 50 of asunaprevir by ~10-fold (wild-type HCV protease IC 50 =6.9±0.6 nM; HCV protease D168E IC 50 =53.5±3.4 nM; HCV protease D168Y IC 50 =214.8±31.9 nM; IC 50 ±s.d.) ( Fig. 4e ). Mutations at position D168 have been previously identified in replicon-based asunaprevir resistance experiments [38] , and the specific D168Y mutation has been observed to arise in hepatitis C patients treated with asunaprevir [39] . Collectively, these results establish that protease PACE in the presence of protease inhibitor drug candidates can very rapidly (1–3 days) reveal clinically relevant mutants that confer strong resistance to the drug candidates, without requiring extensive laboratory or clinical experiments. Previous efforts to use laboratory evolution to study HCV protease inhibitor resistance have relied on time- and labor-intensive approaches such as viral replication in mammalian cell culture or conventional protein evolution methods, which typically require months to complete [22] . By comparison, the continuous evolution of proteases can reveal key resistance mutations in as little as ~1 day of PACE. The speed of PACE and its ability to be multiplexed using many lagoons in parallel, each receiving a different drug candidate, and analysed by high-throughput DNA sequencing of bar-coded lagoon samples, raises the possibility of screening future early-stage hit or lead compounds for their vulnerability to the evolution of drug resistance, before more resource-intensive optimization of in vivo properties or clinical trials take place. Rapid and cost-effective access to drug resistance susceptibility enabled by PACE may enhance the more informed selection of more promising early-stage drug candidates for further development. This technique could also be applied to quickly screen a drug candidate across many distinct genotypic variants of a protease target (such as the six major HCV protease genotypes) to reveal each target variant’s potential to evolve mutations that abrogate the effectiveness of the drug candidate. As HCV patient isolates and replicon assays have already demonstrated differing drug resistance profiles among different HCV genotypes [40] , this capability could also be used to rapidly identify patient-specific drug treatments that are more likely to offer long-term therapeutic effects on patients infected with specific HCV strains, even in the absence of previous data relating strain genotypes to drug effectiveness. The development of protease PACE also expands the scope of PACE to evolve diverse biochemical activities. Previous PACE studies have only evolved RNA polymerases, which have activities that can be directly linked to changes in gIII expression. This study demonstrates how other types of enzymatic activities with no obvious direct connection to gene expression can nevertheless be evolved using PACE by establishing an indirect, but robust, linkage between the activity of interest and gIII expression. The protease PACE system provides a strong foundation for the continuous evolution of proteases with reprogrammed specificities. Previous work on reprogramming the DNA substrate selectivity of T7 RNAP enzymes [25] , [28] , [29] , [30] demonstrated the ability of PACE to rapidly evolve enzymes that accept substrates very different from the native substrate. These reprogramming experiments relied on a ‘stepping-stone’ strategy in which SPs are transitioned between a series of intermediate substrates [28] , and are enhanced by the recent development of modulated selection stringency and negative selection during PACE [30] . In principle these strategies coupled with protease PACE should also enable the continuous evolution of protease enzymes with the tailor-made ability to selectively cleave proteins implicated in human diseases. PA-RNAP gene expression response in vivo All plasmids were constructed by Gibson Assembly 2x Master Mix (NEB); all PCR products were generated using Q5 Hot Start 2x Master Mix (NEB). E. coli strain S1030 (ref. 30 ) were transformed by electroporation with three plasmids: ( i ) a complementary plasmid (CP) that constitutively expresses a PA-RNAP with one of the three protease cut sites ( Supplementary Fig. 2 ), ( ii ) an accessory plasmid (AP, Supplementary Fig. 4 ) that encodes gIII-luciferase (translationally coupled) under control of the T7 promoter and ( iii ) an arabinose-inducible expression plasmid for one of the three proteases (EP, Supplementary Fig. 3 ). The HRV protease gene was purchased as IDT gblocks and cloned into the expression vector. The MBP-TEV fusion protein was amplified by PCR from pRK793 (ref. 41 ). The MBP fusion was necessary for expression and solubility. We deployed a constitutively active HCV protease construct that includes the NS4a cofactor peptide [42] . Cells were grown in 2xYT media to saturation in the presence of antibiotics and 1 mM glucose, then inoculated into 1 ml fresh media containing 1 mM glucose and antibiotics in a 96-well culture plate. After 4.5 h, 150 μl of the cultures were transferred to a black-wall clear-bottom assay plate and luciferase, and OD 600 measurements were taken using a Tecan Infinite Pro plate. The luminescence data were normalized to cell density by dividing by OD 600 . Western blot of PA-RNAP sensor activation E. coli cells transformed with an AP and a CP were grown to log phase, then infected with a 10-fold excess of protease-encoding phage. After 4.5 h, the cells were harvested by centrifugation at 5,000 g for 10 min, and then resuspended in LDS Sample Buffer (Life Technologies). Samples were heated to 95 °C for 5 min and vortexed to shear genomic DNA. Four microlitres of each sample was loaded onto a protein gel electrophoresis system (Bolt gel system, Life Technologies). The blot was performed using a PVDF membrane (iBlot 2 system, Life Technologies). The membrane was blocked with 5% BSA TBST then incubated overnight with the primary antibody (5% BSA, TBST, 1:5,000 anti-T7 RNAP mouse monoclonal, Novagen #70566). The membrane was washed three times, incubated with the secondary antibody (5% BSA, TBST, 1:5,000 donkey anti-mouse, IR-dye conjugate, LI-COR #926-32212) for 60 min, washed three times, then visualized on a LI-COR Odyssey at 800 nm. As seen in Supplementary Fig. 6 , the PA-RNAP sensor is proteolysed to a smaller band of anticipated molecular weight only in the presence of a cognate protease that can cleave the peptide sequence in each PA-RNAP linker. Protease activity-dependent plaque assays Protease phages were cloned using Gibson assembly and the aforementioned expression plasmids as templates. E. coli strain S1030 was transformed by electroporation with an AP and a CP. After the transformed host cells were grown in 2xYT to OD 600 ~1.0, 100 μl of cells was added to 50 μl of serial dilutions of protease-encoding phage. After 1 min, 800 μl of top agar (7 g l −1 agar in 2xYT) was added, mixed and transferred to quarter-plates containing bottom agar (15 g l −1 agar in 2xYT). After overnight incubation at 37 °C, the plates were examined for plaques, which represent zones of slowed growth and diminished turbidity due to phage propagation. PACE propagations and enrichment experiments E. coli strain S1030 was transformed by electroporation with an AP, CP (one for each of the three PA-RNAPs) and a MP ( Supplementary Fig. 7 , Supplementary Table 1 ) encoding arabinose-inducible expression of a dominant-negative mutator variant of dnaQ , wild-type dam and wild-type seqA [43] , [44] , [45] . Starter cultures were grown overnight in 2xYT supplemented with antibiotics and 1 mM glucose to prevent induction of mutagenesis before the PACE experiment. Host cell culture chemostats containing 80 ml of Davis rich media [30] were inoculated with 2 ml of starter culture and grown at 37 °C with magnetic stir-bar agitation. At approximately OD 600 1.0, fresh Davis rich media was pumped in at 80–100 ml h −1 , with a chemostat waste needle set at 80 ml. This fixed dilution rate maintains the chemostat culture in late log phase growth, at which point it can be flowed into lagoons seeded with protease phage (initial titers were ~10 5 p.f.u. ml −1 ). For these experiments, lagoon waste needles were set to maintain a lagoon volume of 15 ml, and host cell cultures were flowed in at 15–17 ml h −1 . Arabinose (10% w/v in water) was added directly to lagoons via syringe pump at 0.7 ml h −1 to induce mutagenesis. Test propagations were conducted with cognate protease phage as well as non-cognate protease phage. Enrichment experiment lagoons were seeded with 1,000-fold excess of non-cognate protease phage. Lagoon samples were sterile-filtered at least every 24 h, and titres were assessed by plaque assay. Plaque assays were performed with S1030 carrying pJC175e, a plasmid that supplies gIII under control of the phage-shock promoter [30] . Mock selections were monitored by PCR of the protease genes with forward primer (BCD582) 5′-TGTTTTAGTGTATTCTTTCGCCTCTTTCGTT-3′ and reverse primer (BCD578) 5′-CCCACAAGAATTGAGTTAAGCCCAATAATAAGAGC-3′ using filtered samples as templates. The distinct sizes of amplicons containing protease genes enabled evaluation of the relative abundance of cognate and non-cognate protease-encoding phage. Uncropped gel images are shown in Supplementary Fig. 8 . Inhibition of PA-RNAP response in host E. coli cells Host cells were prepared by electroporation with an AP and the CP encoding the HCV-site PA-RNAP. We prepared 2xYT media with serial dilutions of inhibitors (danoprevir and asunaprevir, MedChemExpress) from stock solutions made in DMSO and inoculated with a saturated starter culture of host cells. 150 μl cell cultures in a 96-well assay plate were incubated at 37 °C for 1.5 h to allow uptake of inhibitors, then infected with ~10 μl HCV protease phage (multiplicity of infection ~10). After 3 h of incubation at 37 °C, the luminescence of each culture was measured on a Tecan Infinite Pro plate reader and normalized to OD 600 . In the absence of inhibitor, phage-encoded protease will activate the PA-RNAP leading to robust production of luciferase. Relative dose responses to inhibitors compared with control cells without drug were measured in triplicate. Improved mutagenesis plasmid The previous generation of the MP [25] carried four genes: dnaQ926 (ref. 44 ) (a dominant-negative E. coli DNA polymerase III proofreading subunit), umuD’ and umuC (the components of E. coli translesion synthesis polymerase V) and recA730 (an activated recA mutant). The complex of UmuD’ 2 C/RecA730 forms the E. coli mutasome complex, a critical requirement for translesion synthesis across predominantly T-T (6-4) photoproducts and pyrimidine dimers [46] , [47] . As neither type of mutation is predicted to occur commonly during our current PACE experiments, which do not use UV light or chemical mutagens, the genes encoding the mutasome were removed from the MP. To improve the efficiency of mutagenesis, two additional proteins were included on the P BAD transcript: dam (deoxyadenosine methylase) and seqA (a hemimethylated-GATC binding domain), both of which are known mutators when overexpressed in E. coli [43] , [45] . The combination of these three genes yielded higher mutagenesis rates in the presence of arabinose during PACE and resulted in fivefold higher mutagenesis of E. coli chromosomal DNA as assessed by a rifampin resistance assay ( Supplementary Table 1 ). Rifampin resistance assay MG1655 Δ recA E. coli [48] (CGSC#: 12492) cells were transformed with the appropriate MPs and plated on 2xYT/agar plates supplemented with 40 μg ml −1 chloramphenicol and 100 mM glucose to ensure that no induction occurs before the assay. After overnight growth, single colonies were picked into liquid Davis Rich Media [49] supplemented with 40 μg ml −1 chloramphenicol and grown for 12–16 h with vigorous shaking at 37 °C. Cultures were then diluted 1,000-fold in Davis Rich Media and grown until they reached OD 600 =0.5–0.7, at which point they were split into two equal volumes, supplemented with either 100 mM glucose or 100 mM arabinose, and allowed to grow for an additional 24 h. Saturated cultures were serially diluted and plated on 2xYT/agar supplemented with 100 mM glucose with or without 100 μg ml −1 rifampin. After overnight growth, colonies were counted from both plates, and the frequency of resistant mutants was calculated. This measurement been widely used in the literature as a metric of mutagenesis [50] . Evolution of drug resistance in HCV protease using PACE Host cells were the same as those in the HCV test propagation and enrichment experiments. Host cell culture chemostats containing 40 ml of Davis rich media were inoculated with 2 ml of starter culture and grown at 37 °C with magnetic stir-bar agitation. At approximately OD 600 1.0, fresh Davis rich media was pumped in at 50 ml h −1 , with a chemostat waste (outflow) needle set at 40 ml. This adjustment was made to provide enough cell culture to feed two lagoons while also conserving media that contained small-molecule inhibitors. Lagoons were seeded with HCV protease phage and run in duplicate. Again, lagoon waste needles were set to maintain a lagoon volume of 15 ml, and host cell cultures were flowed in at 15–17 ml h −1 . Arabinose (10% w/v in water) was added directly to lagoons via syringe pump at 0.7 ml h −1 to induce the expression of mutagenesis genes on the MP. After 6 h of propagation without any inhibitor, a filtered lagoon sample was taken, and danoprevir was added directly to the chemostat media at 20 μM with 2.5% DMSO to enhance solubility. A final time point was taken after 22 additional hours, and titres were measured by plaque assay on strain S1030 carrying pJC175e. For the asunaprevir experiment, samples were taken every 12 h. After 24 h of propagation with no inhibitor, asunaprevir was added directly to the chemostat media at 10 μM with 2.5% DMSO. After an additional 24 h, asunaprevir dosage was increased to 75 μM and 5% DMSO. Titres were measured by plaque assay on strain S1030 carrying pJC175e. High-throughput sequencing of evolved populations Strain S1030 carrying pJC175e was grown to saturation and used to inoculate fresh media. Host cells were infected with phage samples from the above PACE experiments and incubated for 5 h at 37 °C. DNA from infected cells was extracted using miniprep kits to yield concentrated template phage DNA (Epoch Life Science). PCR reactions were performed using Q5 Hot Start 2x Master Mix (NEB) with a set of tiled primers. The PCR product from the first reaction was diluted ten-fold and 1 μl served as the template for the second PCR. The second PCR added Illumina adapters as well as barcodes; PCR products were purified from agarose gel (Qiagen) and quantified using the Quant-IT Picogreen assay (Invitrogen). Samples were normalized and pooled together to create a sequencing library at ~4 nM. The library was quantified by qPCR (KapaBiosystems) and processed by an Illumina MiSeq using the MiSeq Reagent Kit v3 and the 2x300 paired-end protocol. A single paired-end read of 600 bp is sufficient to cover the entire HCV protease gene. Data were analysed in MATLAB using the custom scripts supplied in the Supplementary Software . FASTQ files were automatically generated by the Illumina MiSeq. These files were already binned by sample barcodes and ready for transfer to a desktop computer. Each read was aligned to the wild-type HCV protease gene in the expected orientation using the Smith-Waterman algorithm. Base calls with Q-scores below a threshold of 31 were converted to ambiguous bases, and the resulting ambiguous codons were turned into a series of three dashes for computationally efficient translation. Ambiguous codons were translated into Xs, which were ignored when tabulating allele counts into a matrix. The script automatically cycled through each FASTQ file and saved the resulting allele count matrix in a separate subdirectory. At this stage, matrices for paired-end reads were added together and normalized to yield allele frequencies for each sample. We relied on a wild-type control sample to assess PCR and sequencing bias. For this sample, we calculated the frequency of alleles that were not wild type at each locus to yield the locus-specific error rate. We added 0.01 (1%) to the locus-specific error rate to yield our variant call threshold. The allele frequency matrix for each sample was scanned for mutant alleles above the variant call threshold. Purification and in vitro assays of evolved HCV variants HCV protease variants were subcloned by Gibson assembly out of the phage genome and into the previously mentioned EP. EPs were transformed into NEB BL21 DE3 chemically competent cells. Starter cultures were grown to saturation, and 2 ml was used to inoculate 500 ml LB. At OD 600 =0.6, cultures were transferred to 20 °C and induced with 0.5% arabinose for 6 h. Cells were harvested by centrifugation at 5,000 g for 10 m, and resuspended in lysis/bind buffer (50 mM Tris-HCl pH 8.0, 500 mM NaCl, 10% glycerol, 5 mM imidazole). Cells were lysed by sonication for a total of 2 min, and then centrifuged for 20 min at 18,000 g to clarify the lysate. Supernatant was flowed through 0.2 ml His-pur nickel resin spin columns that were equilibrated with binding buffer (Pierce-Thermo). Resin was washed with four column volumes of wash buffer (50 mM Tris–HCl pH 8.0, 500 mM NaCl, 10% glycerol, 20 mM imidazole). HCV protease was eluted in four column volumes of 50 mM Tris-HCl pH 8.0, 500 mM NaCl, 10% glycerol, 200 mM imidazole. Samples were further purified by size exclusion chromatography on a SuperDex 75 10/300 GL column (GE Healthcare). Size exclusion was performed in 50 mM Tris–HCl pH 8.0, 100 mM NaCl, 10% glycerol, 1 mM DTT. Protein concentrations were determined by UV 280 on a Nanodrop machine and calculated using an extinction coefficient of 19,000 cm −1 M −1 and a molecular weight of 23 kDa. In vitro assays were performed using the commercial HCV RET Substrate 1 (Anaspec), an internally quenched probe that fluoresces on proteolytic cleavage, according to the manufacturer’s instructions. Protease and inhibitors were incubated in assay buffer at room temperature for 5 m before addition of substrate. Fluorescence was measured every 30 s for 20 m by a Tecan Infinite Pro plate reader (excitation/emission=355 nm/495 nm). Assays were performed at 30 °C with 40 nM protease, 7.5 μM substrate and varying concentration of inhibitors in a final volume of 100 μl per well in black-wall clear-bottom assay plate. The assay buffer contained 50 mM Tris HCl pH 8.0, 100 mM NaCl, 20% glycerol, 5 mM DTT. Assays were performed in triplicate, and initial reaction velocities were calculated and normalized to controls without inhibitor. The data were fit to the Hill Equation using Igor Pro with base and max parameters fixed at one and zero, respectively. The resulting fits yielded IC 50 values and s.d. of the estimate. How to cite this article: Dickinson, B. C. et al. A system for the continuous directed evolution of proteases rapidly reveals drug-resistant mutations. Nat. Commun. 5:5352 doi: 10.1038/ncomms6352 (2014).